Fine structure constant and quantized optical transparency of plasmonic nanoarrays Optics is renowned for displaying quantum phenomena. Indeed, studies of emission and absorption lines, the photoelectric effect and blackbody radiation helped to build the foundations of quantum mechanics. Nevertheless, it came as a surprise that the visible transparency of suspended graphene is determined solely by the fine structure constant, as this kind of universality had been previously reserved only for quantized resistance and flux quanta in superconductors. Here we describe a plasmonic system in which relative optical transparency is determined solely by the fine structure constant. The system consists of a regular array of gold nanoparticles fabricated on a thin metallic sublayer. We show that its relative transparency can be quantized in the near-infrared, which we attribute to the quantized contact resistance between the nanoparticles and the metallic sublayer. Our results open new possibilities in the exploration of universal dynamic conductance in plasmonic nanooptics. There exist only a handful of examples where a measurable property of a physical system is given by a combination of universal constants, for example, quantized resistance [1] , [2] and flux quanta in superconductors [3] , both of which require low temperatures and sophisticated equipment to be investigated. Therefore, it came as a surprise that the dynamic conductance of graphene is determined solely by universal constants [4] , [5] , and, consequently, graphene's absorption in the near-infrared is determined by the fine structure constant [6] , [7] , α . This behaviour was generalized later to any two-dimensional (2D) electronic system with a symmetric homogeneous spectrum [8] where absorption was shown to be quantized in units of πα . Surprisingly, the dynamic conductance G d is different from the conductance quantum G 0 =2 e 2 / h observed in quantum point contacts [1] , [2] (also given by universal constants). The existence of the universal dynamic conductance and the quantized optical transparency of graphene observable at room temperature attracted a lot of interest from researchers in different fields, such as optics, solid state physics and electronics. Here we report another example of quasi-2D systems in which relative optical transparency is quantized in units of πα because of quantization of the dynamic conductance. We show that plasmonic nanoarrays fabricated on a thin metallic sublayer can absorb light in a universal quantized manner. We attribute this quantization to the quantized contact resistance induced by plasmonic near-fields. Our work opens a new direction in studying quantum effects in plasmonic optics. Sample design The studied plasmonic system consists of a high-quality regular array of gold nanoparticles (nanopillars) fabricated on a thin metallic sublayer ( Fig. 1a ). The fabrication and measurement procedures are described in Methods. It is worth noting that the sizes of the nanopillars should be uniform over the whole sample and the thickness of natural oxide of the sublayer should be as small as possible and uniform. Similar regular high-quality arrays have been used to realize ultra-narrow plasmonic resonances [9] , [10] , nanotweezing [11] , optomagnetic [12] , [13] and negative index metamaterials [14] , [15] . 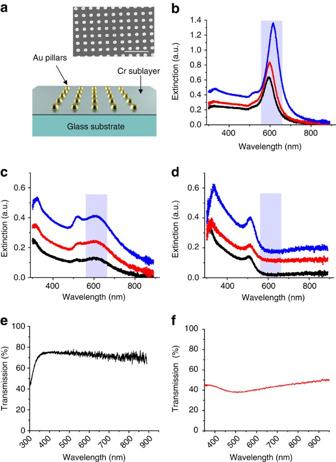Figure 1: Schematics and extinction spectra of plasmonic nanoarrays. (a) Bottom panel: the general design of an array. Top panel: a typical SEM micrograph of a sample. Scale bar is 1 μm. (b–d) Relative extinction spectra for nanopillar arrays with an average diameter ofd=100 nm (black), 110 nm (red) and 130 nm (blue) fabricated on a glass substrate, (b), a glass substrate with a 5-nm Ti sublayer, (c), a glass substrate with a 5-nm Cr sublayer, (d). The array period for the shown spectra is 320 nm. The blue strip marks the LPR region. (e) Absolute light transmission through the 5 nm Ti sublayer deposited on a glass substrate. (f) Absolute light transmission through the 5 nm Cr sublayer on a glass substrate. Figure 1: Schematics and extinction spectra of plasmonic nanoarrays. ( a ) Bottom panel: the general design of an array. Top panel: a typical SEM micrograph of a sample. Scale bar is 1 μm. ( b–d ) Relative extinction spectra for nanopillar arrays with an average diameter of d =100 nm (black), 110 nm (red) and 130 nm (blue) fabricated on a glass substrate, ( b ), a glass substrate with a 5-nm Ti sublayer, ( c ), a glass substrate with a 5-nm Cr sublayer, ( d ). The array period for the shown spectra is 320 nm. The blue strip marks the LPR region. ( e ) Absolute light transmission through the 5 nm Ti sublayer deposited on a glass substrate. ( f ) Absolute light transmission through the 5 nm Cr sublayer on a glass substrate. Full size image Quantized relative transparency of plasmonic nanoarrays Figure 1b shows typical relative optical extinction spectra of the studied nanopillar arrays on a glass substrate for different average sizes of the pillars (at a fixed height of the pillars h =90 nm, and the period of the square lattice a =320 nm) obtained after a wet-etch of the Cr layer. The spectra have been normalized by the light transmission measured outside the arrays, as described in Methods. The nanopillars demonstrate pronounced localized plasmon resonance (LPR) at 600 nm (the LPR region is marked by blue colour), a small peak at 520 nm (which we believe is related to the real part of interband permittivity modified by the presence of the Drude contribution [16] ; for analysis, ref. 15 ) and a broad interband increase of absorption in the ultraviolet range [16] . The presence of the thin metallic sublayer (covered by a naturally formed oxide) under the nanoparticles suppresses the main plasmonic resonance [17] ( Fig. 1c, d ). A less conductive 5 nm sublayer of Ti ( Fig. 1c ) suppresses LPR to a lesser extent than a more conductive 5 nm sublayer of Cr ( Fig. 1d ). At the same time, the presence of the metallic sublayer increases both the interband peak and the interband shoulder in the violet part of the spectrum. For completeness, we show the absolute light transmission through a 5-nm layer of Ti ( Fig. 1e ) and a 5-nm layer of Cr ( Fig. 1f ) deposited on a glass substrate, measured outside the nanopillar arrays and used for the normalization of the spectra. Figure 1e,f can be used to restore the absolute light transmission through the samples. We observed two unexpected features in the measured spectra for samples with the chromium sublayer ( Fig. 1d ). First, the main LPR at the wavelength of 600 nm is completely suppressed, even though the Cr layer is just 5 nm thick. Second, the relative optical extinction of the arrays tends to some constant non-zero values at the near-infrared wavelengths (about 900 nm), where the original LPRs of Figure 1b are not excited. It is these constant values that constitute the main result of our article. Surprisingly, these values are quantized in units of πα when plotted as the relative light transmission. (The relative transmission represents a change of the light transmission induced by the presence of the nanopillars; compare this with ref. 6 .) 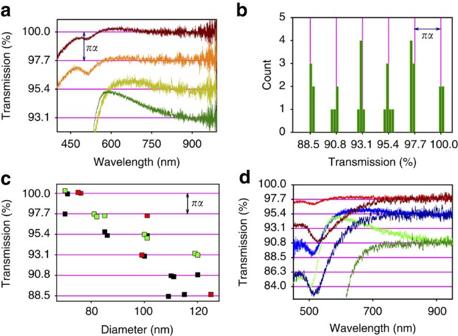Figure 2: Relative optical transmission spectra of arrays fabricated on a 5-nm Cr sublayer. (a) Relative optical transmission measured under normal incidence for nanoarrays with the following parameters: perioda=400 nm and the average pillar diameterd=75 nm (maroon);a=320 nm,d=70 nm (orange);a=320 nm,d=100 nm (yellow);a=320 nm,d=115 nm (green). (b) Histogram of relative optical near-infrared transmission. (c) Near-infrared relative transmission as a function of the nanopillar diameter and the array period: green squares correspond toa=500 nm; red squares:a=400 nm; black squares:a=320 nm. (d) Comparison of the relative transmission for arrays witha=320 nm in the air (bright curves) and in water (dark curves):d=70 nm (red);d=85 nm (blue);d=105 nm (green). Figure 2a shows the relative transmission spectra of four samples measured in the wavelength range of 400–1,000 nm. One can clearly see that the relative transmission for the nanopillar arrays with the Cr sublayer at normal light incidence in the near-infrared tends to constant quantized values Abs = nπα (as the contribution of the pillars to the sample reflection is very small (see below), we assume that in the near-infrared Abs =1– t , where t is the relative transmission). The quantization is especially pronounced for small n . Figure 2: Relative optical transmission spectra of arrays fabricated on a 5-nm Cr sublayer. ( a ) Relative optical transmission measured under normal incidence for nanoarrays with the following parameters: period a =400 nm and the average pillar diameter d =75 nm (maroon); a =320 nm, d =70 nm (orange); a =320 nm, d =100 nm (yellow); a =320 nm, d =115 nm (green). ( b ) Histogram of relative optical near-infrared transmission. ( c ) Near-infrared relative transmission as a function of the nanopillar diameter and the array period: green squares correspond to a =500 nm; red squares: a =400 nm; black squares: a =320 nm. ( d ) Comparison of the relative transmission for arrays with a =320 nm in the air (bright curves) and in water (dark curves): d =70 nm (red); d =85 nm (blue); d =105 nm (green). Full size image Properties of quantization To check this unexpected quantization, we fabricated more than 50 square arrays with different periods ranging from 320 nm to 500 nm, different nanopillar diameters, ranging from 70 nm to 140 nm, and different thicknesses of the chromium sublayer (5 and 7 nm). We found that, whenever the relative light transmission of a sample tends to a constant value in the near-infrared, the relative sample absorption in the near-infrared region is quantized in units of πα . Figure 2b shows the histogram of the near-infrared limit of the relative light transmission for more than 30 samples in which a near-infrared plateau in the transmission has been observed. We clearly see that indeed the relative light transmission in the near-infrared is changing in steps of πα ( Fig. 2b ). The correlation between the quantized transmission and the pillar diameter and array period is shown in Figure 2c . It is worth stressing that the quantized relative transmission is observed well outside the LPR of the array (500–700 nm). To elucidate the nature of the phenomenon, we measured the relative transmission of our structures placed in water and in glycerol. Although the ambient liquid did affect the sample transmission spectra in the visible region, the near-infrared light transmission was still quantized as demonstrated in Figure 2d that shows the relative light transmission spectra for three different arrays measured in air (bright colours) and in water (dark colours) as an example. Array reflection and treatment of samples For small quantization numbers n , the relative transmission of the studied arrays is close to 100%. This implies that an extra reflection generated by the nanopillars is small. Indeed, we measured the reflection from our nanoarrays and found that the difference in the reflection from the sample and the substrate was very small, which implies that studied plasmonic nanoarrays do not reflect much extra light as compared with the substrate ( Fig. 3a ). Hence, the absorption in the nanopillar array can be found from the relative transmission spectrum. 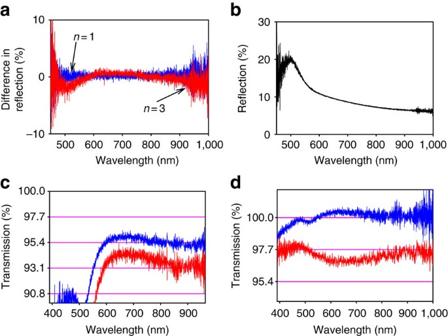Figure 3: Reflection and transmission spectra. (a) Reflection spectra (the difference in reflection between the sample and the substrate) measured under normal incidence on samples that showed quantization plateaus withn=1 (the period of the nanoarraya=500 nm and the average size of the nanopillars isd=80 nm) andn=3 (a=320 nm,d=85 nm). (b) Absolute reflection from an area outside plasmonic nanoarrays fabricated on a substrate covered with a 5 nm Cr layer. (c) Relative light transmission through an array with the average pillar diameterd=100 nm and the lattice perioda=320 nm before (blue) and after (red) 4-hour-illumination with a 100 W Hg lamp. (d) The relative light transmission for an array withd=72 nm,a=500 nm before (blue) and after (red) annealing at 500 °C for 4 h in nitrogen atmosphere. For completeness, Figure 3b shows the absolute reflection from the substrate covered with a 5-nm Cr sublayer measured outside the nanopillar array. Figure 3: Reflection and transmission spectra. ( a ) Reflection spectra (the difference in reflection between the sample and the substrate) measured under normal incidence on samples that showed quantization plateaus with n =1 (the period of the nanoarray a =500 nm and the average size of the nanopillars is d =80 nm) and n =3 ( a =320 nm, d =85 nm). ( b ) Absolute reflection from an area outside plasmonic nanoarrays fabricated on a substrate covered with a 5 nm Cr layer. ( c ) Relative light transmission through an array with the average pillar diameter d =100 nm and the lattice period a =320 nm before (blue) and after (red) 4-hour-illumination with a 100 W Hg lamp. ( d ) The relative light transmission for an array with d =72 nm, a =500 nm before (blue) and after (red) annealing at 500 °C for 4 h in nitrogen atmosphere. Full size image We also studied the change in the light transmission through the sample after it was left under intense light illumination. We found that this procedure did not change the transmission spectra for all but one sample, in which the near-infrared transmission decreased by πα , see Figure 3c . To check whether atom migration had a role in the observed phenomenon, we annealed samples at 500 °C for 4 h in nitrogen atmosphere. This resulted in a decrease in the relative transmission for all samples. The quantization plateaus were still observed but the accuracy of quantization was not as good as for freshly fabricated samples. Figure 3d provides an example of the decrease in the relative transmission for a sample that originally showed 100% relative transmission at the near-infrared frequencies. The physics of modification of the extinction spectra shown in Figures 1b–d is not difficult to understand. Indeed, it is known that an electromagnetic response of a plasmonic array can be modelled by equivalent inductor–capacitor coupled circuits [18] . 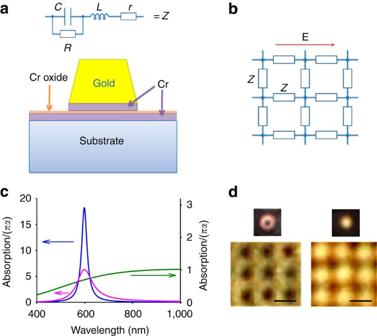Figure 4: Equivalent nanocircuits. (a) Schematics of an individual nanopillar (bottom) and a corresponding electrical nanocircuitZ(top). HereL,Candrrepresent inductance, capacitance and resistance of the nanopillar andRis the shunt resistance. (b) A nanocircuit mesh equivalent to the studied plasmonic nanoarrays. The red arrow represents an electric field E. (c) Relative optical absorption of the nanocircuit mesh for an infinite shunt resistance,R=∞, (blue),R=230kΩ (pink) andR=16.4 kΩ (green). Absorption of the array was calculated using the following parameters (evaluated at visible light frequencies):L=6.3×10−12H,C=1.6×10−20F,r=900 Ω. (d) Dark field images of an individual nanopillar (top) and 3×3 area (bottom) of arrays fabricated on a Cr sublayer (left) and a glass substrate (right). The black scale bars correspond to 500 nm. Array parameters area=500 nm,d=100 nm. Figure 4a shows the schematics of the nanopillar design and a possible equivalent nanocircuit for one nanopillar. Here L and C represent the inductance and capacitance of the resonance circuit (where the contributions from both the individual nanopillar and from the near-field coupling are taken into account); r is the resistance that defines the quality of LPR and R is the shunt resistance produced by the metallic sublayer. It is this shunt resistance that leads to the suppression of LPR shown in Figure 1c–d . Indeed, the studied plasmonic nanoarrays can be modelled by a square mesh of nanocircuits, where each nanocircuit has identical overall impedance Z ( Fig. 4a,b ). When an electric field E is applied parallel to the structure ( Fig. 4b ), simple calculations show that the 2D nature of the array leads to a curious conclusion that the energy losses per unit area do not depend on the period of the lattice and are equal to ( Supplementary Discussion ). Therefore, the relative absorption of an electromagnetic wave of normal incidence can be found as where c is the speed of light ( Supplementary Discussion ). Equation (1) provides a qualitative explanation for the changes in the extinction spectra induced by the presence of the metallic sublayer. When nanopillars are fabricated on a glass substrate, the shunt resistance R is infinite and eq. (1) yields the resonance absorption shown in Figure 4c by the blue line. For a finite and large shunt resistance R , the resonance curve becomes wider and LPR is suppressed, as shown by the pink line in Figure 4c . The suppression increases for a smaller value of the shunt resistance. In this case, the relative absorption tends to a constant value in the near-infrared limit (far from the LPR). As a result, the near-infrared limit of the relative absorption is quantized Abs ~ nπα when the shunt resistance is quantized as shown by the green line for n =1, in Figure 4c . The dynamic conductance of a nanopillar array due to the shunt resistance (2) is given by We put forward a hypothesis that the observed quantization of the relative light transmission through the nanopillar arrays is due to the quantized shunt resistance. The main contribution to the shunt resistance comes from a thin layer of Cr oxide [19] that normally covers the chromium sublayer and produces a tunnel barrier for electrons. (The presence of an extremely thin tunnel barrier and a thin layer of Cr make the finite element analysis of the studied system quite tricky; Supplementary Discussion .) The tunnel resistance due to the natural chromium oxide is large (more than several megaohm) and not quantized. However, the strongly enhanced electromagnetic fields near the studied gold nanoparticles (produced by plasmons) can induce breakdown of the tunnel barrier at the perimeter of the nanopillar base (where the plasmonic near-fields are maximally enhanced). Such breakdown is usually caused by electromigration [20] , [21] , [22] and/or defects [23] , [24] . It is known that the contact resistance of a narrow breakdown/contact channel is quantized [25] , [26] . The dependence of the strength of electromagnetic fields near the edges of a nanopillar on its diameter and the array period would affect electromigration and result in variations in breakdown channels. This could provide an explanation for the transmission plateau dependence on array parameters as shown in Figure 2c . The accuracy of quantization is dramatically improved by averaging of the shunt resistance over the whole array owing to the central limit theorem. (The increase in quantization accuracy for a high-quality homogeneous array with independent and identically distributed random resistances could be roughly evaluated as 1/√ N , where N is the number of illuminated pillars in the array.) Therefore, we speculate that the breakdown in the tunnel barrier results in a set of quantum point channels produced by migrating gold atoms with quantized where n depends on the geometrical properties of the array. The problem of ensemble averaging of the Joule losses in a regular nanoarray, where the breakdown channels are distributed along the perimeter of a nanopillar, is quite complicated. In the Supplementary Discussion , we propose arguments in favour of a heuristic ensemble averaging of the shunt resistance as that agrees with equation (2). A further experimental argument supporting our hypothesis can be found in the dark field images of the arrays. Figure 4d shows the dark field images of the nanoparticles produced on a Cr sublayer and on a bare glass substrate. One can see that nanopillars on a glass substrate scatter light mostly by the plasmonic mode of LPR resulting in the dot-like images of the nanopillars. In contrast, nanopillars fabricated on a Cr sublayer scatter light mostly at their perimeter (where the shunt resistance is active) resulting in the characteristic ring-like images of the nanopillars. It is worth adding that no quantization of light absorption was observed for plasmonic nanoarrays fabricated on a substrate where the metallic sublayer was strongly oxidized. For these samples, the main plasmonic resonance of the arrays was not suppressed by the metallic sublayer and we did not find a quantized plateau in the relative near-infrared light transmission. This again indicates that the breakdown of the tunnel barrier formed by the natural oxide on a metallic sublayer is indeed responsible for the observed quantization. Figure 4: Equivalent nanocircuits. ( a ) Schematics of an individual nanopillar (bottom) and a corresponding electrical nanocircuit Z (top). Here L , C and r represent inductance, capacitance and resistance of the nanopillar and R is the shunt resistance. ( b ) A nanocircuit mesh equivalent to the studied plasmonic nanoarrays. The red arrow represents an electric field E. ( c ) Relative optical absorption of the nanocircuit mesh for an infinite shunt resistance, R =∞, (blue), R =230kΩ (pink) and R =16.4 kΩ (green). Absorption of the array was calculated using the following parameters (evaluated at visible light frequencies): L =6.3×10 −12 H, C =1.6×10 −20 F, r =900 Ω. ( d ) Dark field images of an individual nanopillar (top) and 3×3 area (bottom) of arrays fabricated on a Cr sublayer (left) and a glass substrate (right). The black scale bars correspond to 500 nm. Array parameters are a =500 nm, d =100 nm. Full size image To conclude, we have demonstrated a simple system—a regular array of gold nanopillars fabricated on a chromium sublayer—in which relative optical transparency depends solely on the universal constants and shows unexpected quantization in the near-infrared region. Although the exact nature of the quantization is not yet clear, we suggest that it is related to the quantized shunt resistance between the nanopillars and the metallic sublayer. Our results open new possibilities in studies of the universal optical conductance in plasmonic optics [27] , [28] . Fabrication of nanoarrays High-quality regular, uniform square arrays of gold nanoparticles were produced by e-beam lithography (LEO-RAITH) on a glass substrate covered with a metallic sublayer. The sublayer (5–7 nm) was deposited using Moorfield electron beam evaporation system. The substrate was covered with resist immediately after the sublayer deposition to minimize the thickness of the natural oxide layer. (In samples with a thick oxide layer the main plasmonic resonance of the nanoarrays was not suppressed by the metallic sublayer and we did not observe quantization of the light transmission.) A double-layer resist was used to improve lift-off (80 nm of 495kD PMMA cast from a 3-wt% solution in anisole for the bottom resist layer and 50 nm of 950 kD PMMA cast from a 2-wt% solution in anisole for the top layer). After lithography, we deposited a 5-nm layer of Cr (to improve adhesion) and 90 nm Au by electron beam evaporation, followed by lift-off. The studied arrays of gold nanopillars had periods from 320 nm to 500 nm, average pillar diameters 70–140 nm. A typical size of an array was 0.2×0.2 mm 2 . The samples on a bare glass substrate were obtained from the samples fabricated on a 5-nm Cr sublayer (routinely used to avoid charging during electron beam lithography) in which the Cr sublayer has been wet-etched after fabrication. Optical measurements Optical measurements were performed using USB2000 and USB4000 fibre optic spectrometers. A xenon lamp was used to produce a collimated beam of white light 5 mm in diameter. The beam was focused by a lens with a numerical aperture of 0.1 so that the spot size on the sample was about 50 μm. Transmitted light was collected by a multimode fibre of 400 μm diameter placed immediately after the sample. The relative transmission spectrum was obtained as a ratio of the spectrum measured on the sample to that measured through the substrate (including the metallic sublayer) in the vicinity of the sample. How to cite this article: Kravets, V.G. et al . Fine structure constant and quantized optical transparency of plasmonic nanoarrays. Nat. Commun. 3:640 doi: 10.1038/ncomms1649 (2012).